An earthquake gap south of Istanbul Over the last century the North Anatolian Fault Zone in Turkey has produced a remarkable sequence of large earthquakes. These events have now left an earthquake gap south of Istanbul and beneath the Marmara Sea, a gap that has not been filled for 250 years. Here we investigate the nature of the eastern end of this gap using microearthquakes recorded by seismographs primarily on the Princes Islands offshore Istanbul. This segment lies at the western terminus of the 1999 Mw7.4 Izmit earthquake. Starting from there, we identify a 30-km-long fault patch that is entirely aseismic down to a depth of 10 km. Our evidence indicates that this patch is locked and is therefore a potential nucleation point for another Marmara segment earthquake—a potential that has significant natural hazards implications for the roughly 13 million Istanbul residents immediately to its north. The North Anatolian Fault Zone (NAFZ) is the most active strike-slip fault in Europe and Asia Minor. It acts as the boundary between the Anatolian and Eurasian tectonic plates [1] . This fault has produced a series of large and devastating earthquakes during the 20th century, starting in the west with the 1912 Ganos earthquake and followed in 1939 by the Erzincan earthquake in eastern Anatolia. The locations of these disastrous events have since then systematically propagated westwards towards Istanbul [2] , [3] ( Fig. 1a ). The two most recent earthquakes, both M >7, occurred in 1999, near Izmit and Düzce, to the east of Istanbul. The Izmit event appears to have produced increased seismic activity along the part of the NAFZ that lies immediately south of Istanbul and below the Sea of Marmara [4] . Further to the west, where the NAFZ comes back on land, lies the similar magnitude ( M s ∼ 7.3) 1912 Ganos earthquake rupture segment. The Marmara part of the NAFZ thus appears to represent an earthquake-deficit zone. This zone is as much as 150 km long and is the only part of the NAFZ that has not produced a significant event during last century’s earthquake series. 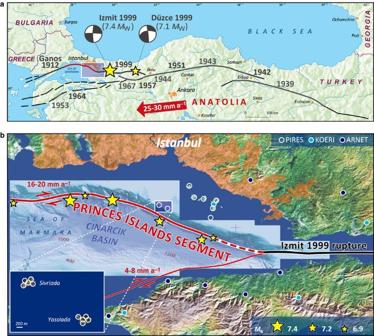Figure 1: Tectonic setting of the NAFZ in Turkey and the larger Istanbul region. (a) Location map of the NAFZ in Turkey. The NAFZ extends∼1,500 km from eastern Anatolia to the Aegean Sea in northern Greece. Black lines and years indicate major earthquakes in the past century. The first event occurred in the west in 1912. The subsequent events started in the east in 1939 and then propagated westward. Yellow stars show the epicentres of the Izmit and Düzce earthquakes of 1999. The red line indicates the segment not ruptured during this series. It lies below the Sea of Marmara and has the potential for aM7.4 earthquake. The red arrow indicates the average annual movement of the Anatolian plate with respect to Eurasia as derived from GPS measurements. The shaded rectangle marks the area of our investigation. (b) The eastern Sea of Marmara region, including the population centre of Istanbul with its >13 million inhabitants. The Princes Islands segment, shown by the bold red line, is the eastern part of the current Marmara seismic gap. The thin red line shows the location of the Armutlu fault. The black line marks the observed rupture zone of the 1999 Izmit event, while the dashed red line indicates its potential link with the Princes Islands segment. Yellow stars mark estimated epicentres of major earthquakes along the Princes Islands segment during the last 2,000 years6,21. White circles mark locations of the PIRES network—the inset showing the two sub-arrays within 2–3 km distance to the fault. Blue and black dots are selected stations of the regional Kandilli Observatory and Earthquake Research Institute (KOERI) and ARNET networks, respectively. Bathymetry is shown for selected areas surrounding the Princes Islands and Cinarcik Basin areas10. Figure 1: Tectonic setting of the NAFZ in Turkey and the larger Istanbul region. ( a ) Location map of the NAFZ in Turkey. The NAFZ extends ∼ 1,500 km from eastern Anatolia to the Aegean Sea in northern Greece. Black lines and years indicate major earthquakes in the past century. The first event occurred in the west in 1912. The subsequent events started in the east in 1939 and then propagated westward. Yellow stars show the epicentres of the Izmit and Düzce earthquakes of 1999. The red line indicates the segment not ruptured during this series. It lies below the Sea of Marmara and has the potential for a M 7.4 earthquake. The red arrow indicates the average annual movement of the Anatolian plate with respect to Eurasia as derived from GPS measurements. The shaded rectangle marks the area of our investigation. ( b ) The eastern Sea of Marmara region, including the population centre of Istanbul with its >13 million inhabitants. The Princes Islands segment, shown by the bold red line, is the eastern part of the current Marmara seismic gap. The thin red line shows the location of the Armutlu fault. The black line marks the observed rupture zone of the 1999 Izmit event, while the dashed red line indicates its potential link with the Princes Islands segment. Yellow stars mark estimated epicentres of major earthquakes along the Princes Islands segment during the last 2,000 years [6] , [21] . White circles mark locations of the PIRES network—the inset showing the two sub-arrays within 2–3 km distance to the fault. Blue and black dots are selected stations of the regional Kandilli Observatory and Earthquake Research Institute (KOERI) and ARNET networks, respectively. Bathymetry is shown for selected areas surrounding the Princes Islands and Cinarcik Basin areas [10] . Full size image Given the annual dextral motion of 23–24 mm a −1 across the Sea of Marmara [5] , this ‘Marmara Earthquake Zone’ may have accumulated a slip deficit of more than 5 m since its last earthquake in 1766. Recent estimates indicate a 35–70% probability for the occurrence of a M >7 earthquake somewhere along it by 2034 (ref. 6 ). Unfortunately its eastern half is close to central Istanbul. Owing to a likely redistribution of post-seismic stress after the 1999 Izmit earthquake, there are suggestions that this eastern part of the Marmara Zone—the ‘Princes Islands segment’—is subjected to enhanced stresses [7] , [8] ( Fig. 1b ). There is also a debate on whether the entire Marmara Zone might rupture as a single through-going strike-slip event, or in several en-echelon normal and oblique faulting events. In the latter case, there might be smaller impacts from the ground motion, but a higher potential for tsunami generation owing to ocean floor elevation changes [9] , [10] , [11] . The primary focus of the study presented here is a better understanding of the physical processes acting in and around the Princes Islands segment. This effort is of course given some urgency by the potential for a major earthquake immediately offshore central Istanbul. We investigate the microseismic activity below the eastern Sea of Marmara west of the 1999 Izmit rupture. We report on an earthquake gap along a substantial part of the Princes Island segment offshore Istanbul that is interpreted to be locked and reflecting a potential nucleation point of the pending Marmara M >7 earthquake. A new earthquake hypocenter catalogue The Princes Islands segment has been monitored by a variety of local seismic networks, including our PIRES array, which was installed in 2006 (refs 11 , 12 ). In addition to our own observations, we have included all available data from these networks to achieve the best possible resolution along this part of the NAFZ. These combined networks include small-aperture arrays on two of the Princes Islands, located there with the aim of lowering the event-detection threshold through beam forming. Data from other, non-array, stations were added to improve the focal coverage. As a result of this effort, the completeness magnitude along the Princes Island segment was lowered by at least one unit, from ∼ 2.8 down to about M ∼ 1.8 ( Fig. 2 , Supplementary Fig. S1 , Supplementary Data 1 ). In the time period of 2006–2010, 835 earthquakes were detected and located. For 783 of these, we successfully applied a relative relocation method [13] providing an internal resolution of better than 150 m. This has allowed us to study the spatial and temporal evolution of the current Princes Island segment activity in unprecedented detail, providing a new view of its brittle deformation. 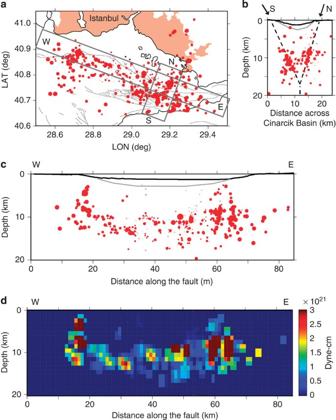Figure 2: Microseismicity along the Princes Islands segment offshore Istanbul. (a) Map view of seismicity during 2006–2010 in the eastern Sea of Marmara region as observed by the PIRES and regional networks. The red location dots are scaled with the magnitudes of their associated earthquakes. The areas enclosed by grey rectangles are shown as enlarged depth sections inbandc. Light grey lines are mapped faults10. (b) Depth section across the Cinarcik Basin revealing the seismicity on the two major fault branches in the eastern Sea of Marmara. In the south the seismicity correlates with the Armutlu fault and in the north with the Princes Islands segment. Surface locations of both faults are indicated by the arrows. The seismicity suggests these faults merge at depth, indicating a single master fault below the seismogenic depth. The dashed lines show the extrapolated faults and their expected merging point at∼18 km depth. (c) Depth section along the Princes Islands segment showing an∼30-km-long and 10-km-deep seismicity gap. The PIRES network is located close to this gap, setting a maximum size of missed events atM∼1.0 (which is slightly lower than the magnitude of completenessMc∼1.8 for the whole catalogue, see electronic supplement). The thick black and grey lines indicate the sea bottom and the base of the Cinarcik Basin, respectively15,16. (d) Cumulative seismic moment release for the 4-year period analyzed in this study along the Princes Islands segment calculated based on the hypocenters shown inc. Figure 2: Microseismicity along the Princes Islands segment offshore Istanbul. ( a ) Map view of seismicity during 2006–2010 in the eastern Sea of Marmara region as observed by the PIRES and regional networks. The red location dots are scaled with the magnitudes of their associated earthquakes. The areas enclosed by grey rectangles are shown as enlarged depth sections in b and c . Light grey lines are mapped faults [10] . ( b ) Depth section across the Cinarcik Basin revealing the seismicity on the two major fault branches in the eastern Sea of Marmara. In the south the seismicity correlates with the Armutlu fault and in the north with the Princes Islands segment. Surface locations of both faults are indicated by the arrows. The seismicity suggests these faults merge at depth, indicating a single master fault below the seismogenic depth. The dashed lines show the extrapolated faults and their expected merging point at ∼ 18 km depth. ( c ) Depth section along the Princes Islands segment showing an ∼ 30-km-long and 10-km-deep seismicity gap. The PIRES network is located close to this gap, setting a maximum size of missed events at M ∼ 1.0 (which is slightly lower than the magnitude of completeness M c ∼ 1.8 for the whole catalogue, see electronic supplement). The thick black and grey lines indicate the sea bottom and the base of the Cinarcik Basin, respectively [15] , [16] . ( d ) Cumulative seismic moment release for the 4-year period analyzed in this study along the Princes Islands segment calculated based on the hypocenters shown in c . Full size image Fault branches merge below seismogenic part of the crust Our refined distribution of hypocenters provides insight into the Princes Island segment seismicity in time and space on a well-resolved scale. For example, we find that the Cinarcik Basin offshore of Istanbul has a wedge-shaped structure, bounded on its north and south sides by different branches of the NAFZ ( Fig. 2b ). The distances between the surface traces of these branches appear to reach a maximum of ∼ 20 km. The fault traces imaged by the seismicity correlate well with those identified from multi-channel seismic profiles showing that the sedimentary fill of the Cinarcik Basin extends as deep as 3–4 km (refs 14 , 15 ). Furthermore, the southward-dipping fault plane for the Princes Islands segment is in good accordance with a recently published model for the formation of the Cinarcik transform basin, in which subsidence is driven by oblique dip-slip on the Princes Islands fault segment [16] . In map view, the inclined nature of each branch results in a diffuse seismicity pattern, seen as an ∼ 10-km-wide northwestern–southeastern striking band. However, band-perpendicular depth sections reveal narrow planes of seismicity inclined towards each other. These planes seem to converge at the lower boundary of the seismogenic zone ( ∼ 18 km) [11] . Characterization of the NAFZ offshore Istanbul The distribution of hypocenters along the Princes Islands segment also contains an ∼ 30-km-long seismically quiet patch, with almost no seismicity above 10 km depth for our observation period ( Fig. 2c ). This 30 × 10 km area is located less than 20 km south of the city centre of Istanbul. It is close to the Princes Islands small-aperture seismic arrays where the detection threshold is lowest, roughly M ∼ 1.0. In contrast, in the same 4-year period, the zones below it, and to its east and west, have hosted most of the observed seismic moment release. This maximum in moment release still corresponds to only one M w 3.5 event for the entire 4-year period ( Fig. 2d ), and includes the zones 5 km to either side of the fault trace. We have considered two end-member hypotheses explaining the seismic silence observed on this portion of the NAFZ. First, it is conceivable that slip along the Princes Island segment occurs entirely by aseismic creep. Second, this segment may be completely locked and thus represents an earthquake or ‘seismic’ gap equivalent to a M ∼ 7 rupture zone. In many similar fault zones around the world, GPS data could be used to sort out these alternatives locally in the near field. In the sea-covered case of the eastern Marmara NAFZ 7 years of regional post-Izmit earthquake GPS data suggest that changes in the regional co-seismic and early post-seismic plate driving stress are negligible [17] , [18] . In other words, either creep or a slip deficit should have been accumulating on this segment in that period. If it was unlocked, numerical models suggest its creep rate would be on the order of 12.8–17.8 mm a −1 —a readily observable amount if appropriate GPS stations were available [19] . Unfortunately, there are few dry places along the entire Marmara part of the NAFZ where GPS measurements could check for this slip. This is especially true for the Princes Islands segment, where no near-fault onshore locations are available to its south. Hence the available data cannot resolve the issue of locked versus creeping behaviour, and we cannot directly rule out fault creep as causing the aseismic patch on this segment (R.E. Reilinger, personal communication). However, historical records report a number of large M >7 earthquakes taking place in the Istanbul region. The last two major events occurred back in 1509 and 1766, fitting a recurrence interval of ∼ 200–250 years (ref. 20 ). Assuming the Princes Island segment was locked before each of these events, they could have nucleated there and then propagated westward along further portions of the Marmara segment. This scenario would result in M >7 earthquakes, similar to those reported in the past centuries. If the Princes Island section is creeping like the central San Andreas fault, then it might show similar responses to regional increases and decreases in seismicity. Along the San Andreas fault system the contrast of highly localized and abundant seismicity versus no or little seismicity on partly creeping or locked segments is striking (e.g. central versus southern SAF Jacinto) is striking and in accordance with surrounding seismic activity, the seismic silence along the Princes Islands segment stands in contrast to the background activity in the broader Izmit-Marmara region. Based on the earthquake catalogue of the Kandilli Observatory and Earthquake Research Institute (KOERI), this activity has increased since the 1999 Izmit event ( Fig. 3 ) [4] . The seismicity rate in the eastern Sea of Marmara region changed from ∼ 7 events per year before to ∼ 14 events per year after the Izmit earthquake (the Izmit aftershocks, which declined according to Omori’s law [21] , were not included in this analysis). This new level of seismicity since ∼ 2002 is consistent with post-1999 stress relaxation processes and enhanced creep rates below the seismogenic part of the crust. 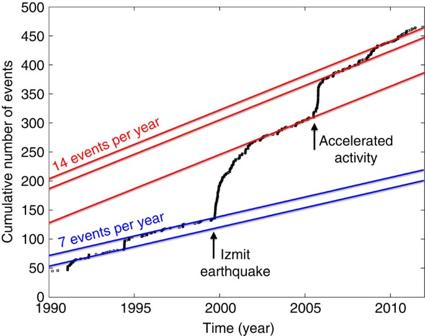Figure 3: Temporal evolution of cumulative seismicity below the eastern Sea of Marmara region. Cumulative number of background earthquakes in the eastern Sea of Marmara region in northwestern Turkey for the time period 1990–2011. The data are from the Kandilli Observatory and Earthquake Research Institute (KOERI) catalogue4. The contributions of the Izmit aftershocks are not considered for calculating the seismicity rates. Further, since the magnitude of completeness was decreasing over this period only events greater thanM=3 are included in this plot (which was the largest completeness magnitude throughout the time period considered). The background seismicity was stable at 7 events per year before the 1999 Izmit earthquake. After 2002, the rate stabilizes at 14 events per year. Accelerated seismicity is observed in 2005 that reflects a local spot of enhanced seismicity but no mainshock–aftershock sequence. Figure 3: Temporal evolution of cumulative seismicity below the eastern Sea of Marmara region. Cumulative number of background earthquakes in the eastern Sea of Marmara region in northwestern Turkey for the time period 1990–2011. The data are from the Kandilli Observatory and Earthquake Research Institute (KOERI) catalogue [4] . The contributions of the Izmit aftershocks are not considered for calculating the seismicity rates. Further, since the magnitude of completeness was decreasing over this period only events greater than M =3 are included in this plot (which was the largest completeness magnitude throughout the time period considered). The background seismicity was stable at 7 events per year before the 1999 Izmit earthquake. After 2002, the rate stabilizes at 14 events per year. Accelerated seismicity is observed in 2005 that reflects a local spot of enhanced seismicity but no mainshock–aftershock sequence. Full size image There is clear evidence for several major ( M >7) earthquakes in the eastern Marmara region throughout the last 2,000 years, the last two being the Izmit 1999 event and the earthquake of 1894, possibly representing its predecessor, both producing notable damage on the Princes Islands [20] , [22] . Considering the historical and current seismicity data, we suggest the available evidence indicates that the Princes Island segment is locked to a depth of ∼ 10 km and accumulating a slip deficit. This is the position we take for the rest of our discussion. Locked fault patches, due to some type of asperity or barrier, are accepted as having fundamental roles in initiation and termination of earthquake ruptures and slip distributions in space and time [23] , [24] , [25] , [26] . Barriers are resistant to failure and do not show microseismicity during the inter-seismic period. When a barrier finally ruptures, surrounding areas can catch up with plate motions, leading to activation of sub-faults and segments [27] . Two recent mega-thrust events, the 2010 Maule offshore-Chile event and the 2011 Tohoku-Oki offshore-Japan event, have confirmed this view and their data are allowing refining understanding M ∼ 9 events. The 2010 Maule event, for example, nucleated in a region of high locking gradient and ended up releasing most of the stress accumulated along its fault plane since the last major event [28] . We suggest that such a scenario may apply to the Princes Island and Marmara segments of the NAFZ. How might an earthquake rupture of the Marmara segment proceed? For example, can temporal changes in seismicity along the Princes Island segment be related to the varying contributions of strike slip and normal faulting in the past? The 1999 Izmit earthquake also showed clear segmentation in space and time [3] , [29] , [30] , [31] , [32] . Propagating eastward, it took just a few seconds for this event to initiate slip on the Karadere segment ( Fig. 4 ). The Izmit rupture terminated at the transition of the Karadere segment to the Düzce Basin. This apparently activated the adjacent Düzce segment 87 days later, resulting in a M 7.1 earthquake, extending the slip zone by another ∼ 40 km further east [33] . The Düzce rupture also fits the scheme of 20- to 40-km-long fault segments failing in a cascade along the NAFZ. Following this scenario to the west of Izmit, activation of the Princes Islands earthquake gap would seem to be still pending ( Fig. 4 ). Furthermore, Coulomb stress models after the Izmit event but before the Düzce event indicate a stress increase at the Düzce and Princes Islands segments [7] , [8] . 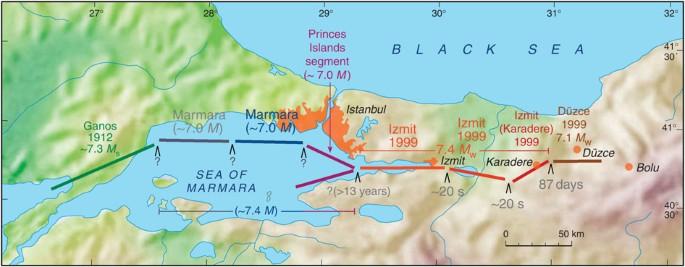Figure 4: Segmentation of the NAFZ in northwestern Turkey. Major NAFZ fault segments in the Marmara and Izmit regions in northwestern Turkey (simplified). Two potential future rupture scenarios and their associated earthquake magnitudes are shown reflecting the activation of the Marmara segment of the NAFZ as one single (∼7.4M) or multiple (∼7.0M) events. Green, orange/red and brown lines mark major fault segments of the Ganos 1912, Izmit 1999 and Düzce 1999,M>7, rupture zones, respectively. The Marmara seismic gap between the Ganos and Izmit zones has not experienced a similar sized event since 1766. The numbers between segment boundaries are observed time delays between the initiations of slip on consecutive segments. Question marks indicate potential segment boundaries beneath the Sea of Marmara. Figure 4: Segmentation of the NAFZ in northwestern Turkey. Major NAFZ fault segments in the Marmara and Izmit regions in northwestern Turkey (simplified). Two potential future rupture scenarios and their associated earthquake magnitudes are shown reflecting the activation of the Marmara segment of the NAFZ as one single ( ∼ 7.4 M ) or multiple ( ∼ 7.0 M ) events. Green, orange/red and brown lines mark major fault segments of the Ganos 1912, Izmit 1999 and Düzce 1999, M >7, rupture zones, respectively. The Marmara seismic gap between the Ganos and Izmit zones has not experienced a similar sized event since 1766. The numbers between segment boundaries are observed time delays between the initiations of slip on consecutive segments. Question marks indicate potential segment boundaries beneath the Sea of Marmara. Full size image The contrast between the increased seismic activity in the eastern Sea of Marmara region since ∼ 2002 and quiescence along the Princes Island segment offshore Istanbul is striking. It adds to the suggestion that this patch in the 150-km-long seismic gap below the Sea of Marmara may be the nucleation point of a future earthquake. The Princes Islands segment may have acted as a barrier to the 1999 Izmit rupture, preventing slip to continue towards Istanbul [34] . These possibilities are important with respect to the segmentation of major ruptures along the NAFZ in northwestern Turkey. With the cascade-like activation of fault segments towards the Istanbul metropolitan region, the Princes Island earthquake gap must be considered to have a substantial impact on the seismic hazard potential for Istanbul. Even though a long-term earthquake catalogue exists for the NAFZ in general and for the Istanbul region in particular, fundamental understanding of the earthquake machine there is still a long way off. Our observation of an earthquake gap in direct vicinity to the Istanbul metropolitan region presented here was made possible through deploying closely spaced seismic stations and small arrays near the fault trace south of the Princes Islands. This improved microseismic monitoring along the Princes Islands segment, west of the Izmit 1999 rupture and southeast of metropolitan Istanbul is highlighting the location of likely rupture nucleation points for the pending Marmara earthquake. It also constrains the maximum size of future events along the Marmara seismic gap in case of cascade behaviour. Our results justify the need of a regional earthquake early warning system for metropolitan Istanbul. Indeed, the observed aseismic portion of the Princes Islands segment might represent a potential high-slip patch in a future earthquake. Precise fault-zone characterization is likewise relevant for determining the directivity of seismic waves approaching Istanbul. Recent modelling of the potential impacts of different earthquake scenarios have shown to substantially improve estimation of the hazards they pose [35] . In similar ways, improved seismic monitoring is expected from current efforts to install a borehole-based seismometer network in the eastern Sea of Marmara region [36] . Following the strategy of the High Resolution Seismic Network on the Parkfield segment of the San Andreas Fault, these stations will provide increasingly better insights into the processes acting on the Princes Island earthquake gap, and thus into the occurrence of large earthquakes in space and time. Earthquake relative relocation To achieve the best hypocentral location resolution of our data set, we have used a waveform-based double-difference relative relocation method [13] . The method uses relative arrival times for events that are close to each other, placing them in precise but relative locations. This suppresses the effect of complex velocity structure on relative locations, as the ray paths of closely located events are almost identical. We improved our initially manually picked differential travel times by using a waveform cross-correlation technique [37] . Consequently, the differential travel times could also be measured much more precisely than absolute arrival times. This also resulted in more precise relative hypocenter locations. So when combined, the double-difference and cross-correlation methods allowed to significantly improve the precision of the event locations relative to each other while the absolute precision of the entire hypocenter catalogue is ∼ 2 km. The relative location precision of events typically ranged between 50 and 150 m, distances that are comparable to the size of their associated source radii. However, we believe that the actual location errors are larger than the covariance-derived error estimates, especially for the event pairs several source-sizes away from each other. Leaving out events too far apart for the correlation and differencing assumptions to be valid, our final hypocenter catalogue of relocated events includes 783 earthquakes ( Fig. 2a , Supplementary Data 1 ). How to cite this article: Bohnhoff M. et al . An earthquake gap south of Istanbul. Nat. Commun. 4:1999 doi: 10.1038/ncomms2999 (2013).